Erythropoietin production in neuroepithelial and neural crest cells during primitive erythropoiesis Erythropoietin (Epo) supports both primitive erythropoiesis in the yolk sac and definitive erythropoiesis in the fetal liver and bone marrow. Although definitive erythropoiesis requires kidney- and liver-secreted Epo, it is unclear which cells produce Epo for primitive erythropoiesis. Here we find neural Epo-producing (NEP) cells in mid-gestational stage embryos using mouse lines that express green fluorescent protein (GFP) under the Epo gene regulation. In these mice, GFP is expressed exclusively in a subpopulation of neural and neural crest cells at embryonic day 9.0 when Epo-deficient embryos exhibit abnormalities in primitive erythropoiesis. The GFP-positive NEP cells express Epo mRNA and the ex vivo culture of embryonic day 8.5 neural tubes results in the secretion of Epo, which is able to induce the proliferation and differentiation of yolk sac-derived erythroid cells. These results thus suggest that NEP cells secrete Epo and might support the development of primitive erythropoiesis. Erythropoietin (Epo) is one of the best-characterized cytokines that stimulates the proliferation and differentiation of erythroid cells [1] . Epo binds to the Epo receptor (EpoR) on the surface of erythroid progenitor (EP) cells and stimulates the proliferation and maturation of progenitor cells via the phosphorylation of EpoR and associated signalling molecules [2] . Tissue hypoxia that is caused by anaemia or altitude sickness induces Epo gene expression in the kidney and liver of adult humans and mice [1] , [3] . This hypoxia-induced Epo gene expression is transcriptionally regulated by hypoxia-inducible transcription factors (HIFs). The first characterized HIF-binding sequence (that is, hypoxia responsive element or HRE) resides in the 3′-region of the Epo gene [4] , [5] , [6] . The first wave of murine erythropoiesis begins in the blood islands of the visceral yolk sac at embryonic day 7.5 (E7.5). This erythropoiesis is referred to as primitive erythropoiesis [7] , [8] . The fetal liver subsequently becomes the principal erythropoietic tissue in late-stage embryos. Around birth, erythropoiesis moves to the bone marrow and spleen [6] . The latter type of erythropoiesis is referred to as definitive erythropoiesis [7] , [8] . Yolk sac-derived erythrocytes express embryonic β-globin (ε y -globin), whereas definitive erythrocytes express adult-type β-globin (primarily β maj -globin) [8] . This shift of erythropoiesis from one tissue to another and the change in globin- gene expression are common features of vertebrate erythropoiesis. Mouse and human definitive erythrocytes in the peripheral blood are enucleated, whereas primitive erythrocytes have a nucleus when they are released from yolk sac and complete their maturation (enucleation) while circulating [9] , [10] . Tissues other than the liver and kidney also secrete Epo, but whether Epo makes critical contributions to non-haematopoietic tissues or cells remains to be clarified [11] , [12] , [13] , [14] , [15] , [16] . In contrast, transgenic complementation rescue analyses of EpoR gene revealed that EpoR expression in non-haematopoietic tissues is dispensable for mouse survival and fertility [17] . Thus, while Epo also has non-haematopoietic functions under pathological or stress conditions, the principal role of Epo is to support erythropoiesis. Epo or EpoR gene knockout mice are lethal at ~E12.5 because of a defect in definitive erythropoiesis [18] . We have identified renal Epo-producing (REP) cells in the interstitial space of the kidney [19] , [20] , [21] . REP cells secrete Epo into the bloodstream where it acts as an endocrine factor for bone marrow EPs [6] , [22] . While adult mouse hepatocytes also produce low levels of Epo, this hepatic Epo production is dispensable for erythropoiesis in adult mice [6] , [23] . In contrast, fetal liver-derived Epo stimulates liver erythropoiesis in a paracrine manner [6] . Importantly, Epo or EpoR gene knockout mice also exhibit an inefficient production of primitive erythrocytes, suggesting that Epo plays important roles in primitive erythropoiesis [18] . However, Epo-producing cells in the early stages of mouse development have not been identified. Therefore, in the present study we address Epo production in early-stage embryos. We observe Epo production in neural and neural crest cells of E8.5–E11.5 embryos. We also determine that this Epo production is able to induce the proliferation and differentiation of yolk sac-derived erythroid cells under ex vivo co-culture conditions. The major source of Epo for primitive erythropoiesis might be a subpopulation of neural and neural crest cells, which we refer to as neural Epo-producing (NEP) cells. The indispensable roles of Epo in primitive erythropoiesis To elucidate the contribution of Epo to primitive erythropoiesis, we analysed an Epo-knockout (Epo-KO or Epo −/− ) mouse line ( Supplementary Fig. S1 ) [20] , [21] . No apparent abnormality was observed in Epo-KO embryos at E8.5 (5–9 somite pair stages (sp); Fig. 1a ) or E9.0 (16–20 sp; Fig. 1a ). Nonetheless, the yolk sacs of Epo-KO mice were moderately and severely anaemic at E10.5 and E11.5, respectively ( Fig. 1a ). We found that Epo-KO embryos died by E12.5 due to anaemia, and this is consistent with the previous observations [18] . 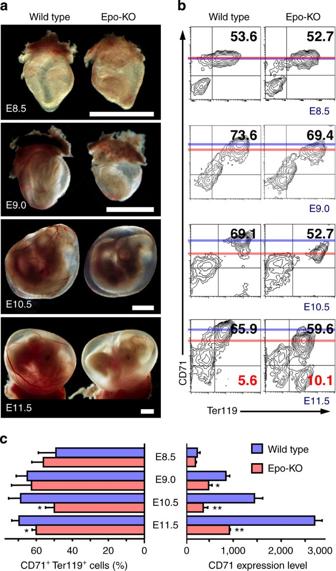Figure 1: Epo is required for primitive erythropoiesis in mouse embryos after E9.0. (a) Whole-mount images of wild-type and Epo-KO embryos at the indicated stages (E8.5, E9.0, E10.5 and E11.5). Scale bars, 1.0 mm. (b) FACS analysis of yolk sac cells from wild-type and Epo-KO embryos at E8.5 (5–9 sp), E9.0 (16–20 sp), E10.5 and E11.5. The relative abundance of the CD71+Ter119+fraction is indicated in each panel as a percentage. The blue and red lines indicate the mean fluorescent intensities of CD71 expression in the Ter119+CD71+fractions of wild-type and Epo-KO embryos, respectively. (c) The relative abundance (left) and CD71 expression levels (right) of the CD71+Ter119+fraction in the yolk sac cells from wild-type and Epo-KO embryos at the indicated stages. FACS data from more than three embryos in each group are presented with s.d. *P<0.05, **P<0.01 when compared with the wild-type controls, based on Student’st-test. Figure 1: Epo is required for primitive erythropoiesis in mouse embryos after E9.0. ( a ) Whole-mount images of wild-type and Epo-KO embryos at the indicated stages (E8.5, E9.0, E10.5 and E11.5). Scale bars, 1.0 mm. ( b ) FACS analysis of yolk sac cells from wild-type and Epo-KO embryos at E8.5 (5–9 sp), E9.0 (16–20 sp), E10.5 and E11.5. The relative abundance of the CD71 + Ter119 + fraction is indicated in each panel as a percentage. The blue and red lines indicate the mean fluorescent intensities of CD71 expression in the Ter119 + CD71 + fractions of wild-type and Epo-KO embryos, respectively. ( c ) The relative abundance (left) and CD71 expression levels (right) of the CD71 + Ter119 + fraction in the yolk sac cells from wild-type and Epo-KO embryos at the indicated stages. FACS data from more than three embryos in each group are presented with s.d. * P <0.05, ** P <0.01 when compared with the wild-type controls, based on Student’s t -test. Full size image To characterize the yolk sac cells of Epo-KO embryos, we conducted flow cytometry analyses. In wild-type yolk sacs, transferrin receptor (CD71) expression in Ter119 + erythroblasts (EBs) gradually increased during embryonic development ( Fig. 1b ), whereas the increase was not so significant for Epo-KO yolk sacs. The CD71 fluorescence intensity was markedly lower in Epo-KO yolk sacs than that in wild-type yolk sacs after E9.0 ( Fig. 1c ). Moreover, the relative abundance of CD71 + Ter119 + cells was decreased in Epo-KO yolk sacs after E10.5 compared with those in wild-type yolk sacs ( Fig. 1c ). These results support our contention that Epo contributes to primitive erythropoiesis and is required for the differentiation of primitive erythroid cells towards the CD71-positive stage in yolk sacs after E9.0. Epo expression in developing neural tissues To our current knowledge, the earliest time of Epo expression is at E9.5 in the liver [24] . However, the impaired primitive erythropoiesis in Epo-KO mice implies that Epo is produced in embryos around E9.0, although Epo-producing tissues or cells have not been identified in early-stage embryos. To identify Epo-producing tissues or cells in mid-gestational stage embryos, we dissected embryos ( Supplementary Fig. S2a–c ) at E8.5 (5–9 sp), E9.5 (22–25 sp) and E10.5, and analysed Epo messenger RNA expression using reverse transcription (RT)–quantitative PCR (qPCR). To our surprise, Epo mRNA was exclusively expressed in the head region at E8.5 ( Fig. 2a ). As Epo mRNA was not detected in samples from whole embryos at E7.5, the head region of E8.5 embryos appeared to be the first Epo-producing tissue during mouse embryogenesis. Epo mRNA expression was detected in the head region and in the fetal liver in E9.5 and E10.5 embryos ( Fig. 2a ) [6] , [24] . The relative Epo mRNA expression level in the head region gradually decreased during development and was undetectable at E11.5, whereas Epo mRNA expression in the fetal liver gradually increased over this period ( Fig. 2a ). 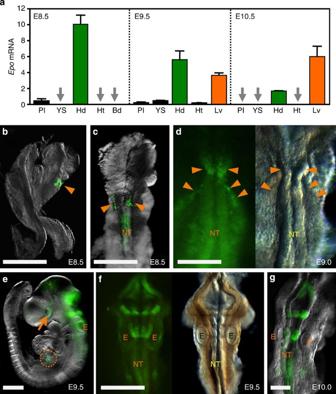Figure 2: Embryonic neural tissues in the mid-gestation embryo transiently express Epo. (a) RT–qPCR analyses ofEpomRNA expression in the placenta (Pl), the yolk sac (YS), the head (Hd), the heart (Ht), the body proper (Bd) and the liver (Lv) of wild-type embryos at E8.5 (5–9 sp), E9.5 (22–25 sp) and E10.5. The data indicate the averages of the relative expression levels with s.d. The levels were normalized usingGapdhmRNA expression levels, and three embryos were analysed in each sample. Note thatEpomRNA expression is detectable in heads (green) and livers (orange) of the embryos. The grey arrows indicate undetectable levels. (b–g) The GFP expression profile in22K-Epo-GFPtransgenic mouse embryos at E8.5 (b,c), E9.0 (d), E9.5 (e,f) and E10.0 (g). GFP-positive cells are observed in or around the neural folds (arrowheads inb–d) at E8.5 and E9.0. Dotted circle, fetal liver; orange arrow, optic vesicle; E, otic vesicle; NT, neural tube. Scale bars, 0.5 mm (b,e,f) and 0.2 mm (c,d,g). Figure 2: Embryonic neural tissues in the mid-gestation embryo transiently express Epo. ( a ) RT–qPCR analyses of Epo mRNA expression in the placenta (Pl), the yolk sac (YS), the head (Hd), the heart (Ht), the body proper (Bd) and the liver (Lv) of wild-type embryos at E8.5 (5–9 sp), E9.5 (22–25 sp) and E10.5. The data indicate the averages of the relative expression levels with s.d. The levels were normalized using Gapdh mRNA expression levels, and three embryos were analysed in each sample. Note that Epo mRNA expression is detectable in heads (green) and livers (orange) of the embryos. The grey arrows indicate undetectable levels. ( b – g ) The GFP expression profile in 22K-Epo-GFP transgenic mouse embryos at E8.5 ( b , c ), E9.0 ( d ), E9.5 ( e , f ) and E10.0 ( g ). GFP-positive cells are observed in or around the neural folds (arrowheads in b – d ) at E8.5 and E9.0. Dotted circle, fetal liver; orange arrow, optic vesicle; E, otic vesicle; NT, neural tube. Scale bars, 0.5 mm ( b , e , f ) and 0.2 mm ( c , d , g ). Full size image To identify which cell types express Epo in the embryonic head region, we next examined transgenic mouse lines that express green fluorescent protein (GFP) under the control of the Epo regulatory region. To this end, we used transgenic mouse lines that carried various bacterial artificial chromosome-based GFP reporter transgenes that we previously established ( Table 1 ; Supplementary Fig. S1 ) [6] , [15] , [19] , [22] . Importantly, it has been shown that GFP fluorescence in these mice faithfully recapitulates the endogenous Epo gene expression profile in adult livers and kidneys. Table 1 Epo-GFP transgene expression in E9.5 embryos. Full size table We analysed seven lines of transgenic mice that carried wt-Epo-GFP , 22K-Epo-GFP or 17KXh-Epo-GFP transgenes [6] , [15] , [19] , [22] and found that all these mice exhibited green fluorescence in rostral neural tissues and liver at E9.5 (22–25 sp) with a conserved expression profile ( Table 1 ). The representative GFP expression patterns in 22K-Epo-GFP transgenic mouse embryos are shown in Fig. 2b–g . In E8.5–E10.0 embryos, green fluorescence was detected in rostral neural tissues, and the expression in the rhombomeres (especially in r1, r3 and r5) was strong ( Fig. 2f,g ). E9.5–E11.5 embryos also expressed GFP in the liver ( Fig. 2e ; Supplementary Fig. S2c,d ). The expression profile and GFP intensity in the transgenic mouse embryos were comparable with the RT–qPCR data, revealing high-level expression in the head region at E8.5 and a decrease in this expression during development. Thus, these results demonstrate that cells in neural tissues of E8.5–E11.5 embryos express Epo. We refer to these cells as NEP cells. Regulatory elements for Epo gene expression in NEP cells To examine cis -acting regulatory elements of the Epo gene using transgenic reporter expression assays, we assessed GFP reporter expression in two bacterial artificial chromosome transgenic mouse lines that carry the wt-Epo-GFP , three lines that carry the 22K-Epo-GFP and two lines that carry the 17KXh-Epo-GFP (transgene structures are shown in Supplementary Fig. S1 ) [15] , [19] , [22] . Transgenic mouse embryos of all seven lines expressed GFP in NEP cells at E9.5 ( Table 1 ), strongly supporting the notion that the GFP reporter expression, and hence Epo gene expression, in NEP cells is reproducible and physiological. We also conclude that the transactivation event that induces Epo gene expression in NEP cells resides within a 32-kb region that spans the 17-kb upstream and 15-kb downstream of the Epo gene ( Supplementary Fig. S1 ). Of the regulatory motifs within this 32-kb region, we have identified important roles such as (i) the GATA-binding motif (5′-GATA) in the proximal promoter [19] and (ii) the HIF-binding motif in the 3′-enhancer (3′-HRE) [6] play. These findings were drawn by using mouse lines that carry the wt-Epo-GFP and its mutant transgene constructs. Taking advantage of these transgenic mouse lines, we examined the contribution of these cis -acting elements to Epo gene expression in NEP cells. Two types of mutations in the 5′-GATA motif in a total of four transgenic mouse lines (two lines for each mutation) were utilized to assess GFP expression in E9.5 embryos. The 5′-GATA motif was not required for GFP expression in NEP cells but was essential to repress ectopic GFP expression in the epidermis ( Table 1 ). Similarly, analyses of 3′-HRE-mutant transgenes ( m3-Epo-GFP ) revealed that 3′-HRE was dispensable for reporter expression in NEP cells ( Table 1 ). These results indicate that the cis -acting regulatory elements for Epo gene expression in NEP cells reside in the 35-kb region but are independent of 5′-GATA and 3′-HRE. Epo-GFP transgene expression in developing neuroepithelium We found that GFP expression in the head region decreased in Epo-GFP transgenic mouse embryos after E10.5, while the fetal liver consistently expressed GFP after E9.5 ( Fig. 3a–d ). Since GFP expression was observed in the neuroepithelium around hindbrain ( Fig. 3a,b ), we conducted immunofluorescent analyses using antibodies against GFP and Sox2, a marker for developing neuroepithelial cells [25] . There are GFP + cell fractions in the neuroepithelium and nuclear staining of Sox2 in the GFP + cells, demonstrating that a part of neural lineage cells express the Epo gene at E9.5 ( Fig. 3e,f ). 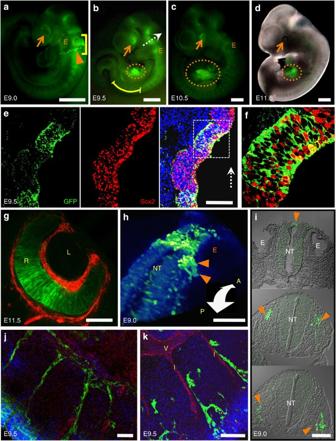Figure 3: The expression of theEpo-GFPtransgenes in mouse embryos. (a–d) GFP expressions in22K-Epo-GFP(a,d) and17KXh-Epo-GFP(b,c) transgenic mouse embryos at E9.0 (a), E9.5 (b), E10.5 (c) and E11.5 (d). Orange arrow, optic vesicle; E, otic vesicle; dotted circle, fetal liver. (e,f) Immunofluorescence of GFP (green) and Sox2 (red) in the transverse section of hindbrain (location is indicated by the dotted arrow inb) from a17KXh-Epo-GFPtransgenic mouse embryo at E9.5. The right panel ofeis a merged image of left (GFP) and middle (Sox2) panels with counterstaining by 4′,6-diamidino-2-phenylindole (DAPI; blue). GFP is expressed in Sox2-positive neuroepithelial cells (f, the higher magnification image of the dotted quadrangle ine). The dotted arrow indicates the dorsal direction. (g) The section of eye (R, retina; L, lens) from a22K-Epo-GFPembryo at E11.5 shows that GFP is expressed in the retina surrounded by CD31+endothelial cells (red). (h) GFP expression in a three-dimensional image of a22K-Epo-GFPembryo at E9.0. A dorsal view of the posterior (P)–anterior (A) axis was obtained using a laser confocal microscope with Amira software. GFP-positive cell clusters (arrowheads) are observed around the otic vesicle (E) and the neural tube (NT). (i) GFP expression in transverse sections around the rostral neural tube (indicated by the yellow line ina) of an E9.022K-Epo-GFPtransgenic embryo. Serial sections are exhibited in a rostral-caudal order (upper-lower). (j,k) GFP expression in the intersomitic space of a17KXh-Epo-GFPtransgenic embryo at E9.5. GFP (green) and CD31 (red) immunofluorescence in sagittal sections of somites (yellow line inb) is shown with counterstaining by DAPI (blue) at low (j) and high (k) magnifications. V, aorta; I, intersomitic artery. Scale bars, 100 μm (e,h–k), 400 μm (a–c,g) and 1.0 mm (d). Figure 3: The expression of the Epo-GFP transgenes in mouse embryos. ( a – d ) GFP expressions in 22K-Epo-GFP ( a , d ) and 17KXh-Epo-GFP ( b , c ) transgenic mouse embryos at E9.0 ( a ), E9.5 ( b ), E10.5 ( c ) and E11.5 ( d ). Orange arrow, optic vesicle; E, otic vesicle; dotted circle, fetal liver. ( e , f ) Immunofluorescence of GFP (green) and Sox2 (red) in the transverse section of hindbrain (location is indicated by the dotted arrow in b ) from a 17KXh-Epo-GFP transgenic mouse embryo at E9.5. The right panel of e is a merged image of left (GFP) and middle (Sox2) panels with counterstaining by 4′,6-diamidino-2-phenylindole (DAPI; blue). GFP is expressed in Sox2-positive neuroepithelial cells ( f , the higher magnification image of the dotted quadrangle in e ). The dotted arrow indicates the dorsal direction. ( g ) The section of eye (R, retina; L, lens) from a 22K-Epo-GFP embryo at E11.5 shows that GFP is expressed in the retina surrounded by CD31 + endothelial cells (red). ( h ) GFP expression in a three-dimensional image of a 22K-Epo-GFP embryo at E9.0. A dorsal view of the posterior (P)–anterior (A) axis was obtained using a laser confocal microscope with Amira software. GFP-positive cell clusters (arrowheads) are observed around the otic vesicle (E) and the neural tube (NT). ( i ) GFP expression in transverse sections around the rostral neural tube (indicated by the yellow line in a ) of an E9.0 22K-Epo-GFP transgenic embryo. Serial sections are exhibited in a rostral-caudal order (upper-lower). ( j , k ) GFP expression in the intersomitic space of a 17KXh-Epo-GFP transgenic embryo at E9.5. GFP (green) and CD31 (red) immunofluorescence in sagittal sections of somites (yellow line in b ) is shown with counterstaining by DAPI (blue) at low ( j ) and high ( k ) magnifications. V, aorta; I, intersomitic artery. Scale bars, 100 μm ( e , h – k ), 400 μm ( a – c , g ) and 1.0 mm ( d ). Full size image We isolated the GFP + cells from the head region of 17KXh-Epo-GFP transgenic mouse embryos at E9.5 using fluorescence-activated cell sorter (FACS; Supplementary Fig. S2e ). RT–qPCR analyses of the isolated cells showed co-expression of neural marker mRNAs ( Sox2 and Nestin ) [25] , [26] with Epo mRNA in NEP cells ( Supplementary Fig. S3a ). Epo-GFP expression was also observed in neuroepithelia of the otic and optic vesicles ( Figs 2e,f and 3a,b ), and the expression was detectable in the retinal neuroepithelium until E11.5 ( Fig. 3g ). These results thus demonstrate that Epo is expressed transiently in a subpopulation of developing neural cells. Strong Epo-GFP expression in a neural crest cell cluster We detected a cell cluster expressing very bright green fluorescence posterior to the otic vesicle in the 17KXh-Epo-GFP and 22K-Epo-GFP transgenic embryos at E9.0 (arrowheads in Figs 2d and 3a,h,i ). The cell cluster formed a line from the dorsal neural tube to the developing heart ( Supplementary Fig. S3b ), which was considered to be a migration stream of cardiac neural crest cells [27] , and the cells seemed to be derived from the initially emerged NEP cells in E8.5 embryos (arrowheads in Fig. 2b,c ). These GFP high cells were observed in all Epo-GFP transgenic mouse lines examined ( Table 1 ). Since Epo is a secreted factor, it is plausible that these GFP high cells dominantly produce Epo among NEP cells. At E9.5, GFP-positive cells were detected in intersomitic spaces ( Fig. 3j,k ). These GFP-positive cells resided posterior to the intersomitic vessels, which were lined with CD31 + endothelial cells ( Fig. 3j,k ). It seems plausible that the close proximity between NEP cells and the vessels ( Fig. 3g,j,k ) is effective for prompt secretion of Epo into the bloodstream. Since trunk neural crest cells migrate into the intersomitic space from dorsal to ventral side of embryos [27] , we conclude that NEP cells consist of a subpopulation of neural crest cells and a subpopulation of neural lineage cells. A subpopulation of neural crest cells produces Epo To further verify that NEP cells include neural crest cells, we crossed the 17KXh-Epo-GFP mice with the neural crest cell-tracer mouse line Wnt1-Cre::Rosa26R-tdTomato ( Supplementary Fig. S3c ) [28] . We found that a subpopulation of tdTomato-positive cells around the neural tube expressed GFP in E9.5 embryos ( Fig. 4a,b ). We conducted similar experiments using two additional neural crest tracer lines of mice, Pax3-Cre::Rosa26R-tdTomato [29] and P0-Cre::Rosa26R-tdTomato [30] . The results demonstrated that GFP-positive cells were partially overlapped with tdTomato-positive cells in these tracer mouse lines ( Supplementary Fig. S3d–i ). 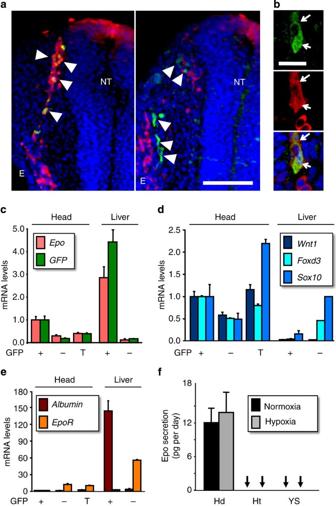Figure 4: A subpopulation of neural crest cells express theEpogene. (a,b) Both GFP (green, arrowheads) and tdTomato (red) expression is detected in transverse sections of the neural tube (NT) from E9.517KXh-Epo-GFP:Wnt1-Cre:Rosa26R-tdTomatoembryos using confocal microscopy. DAPI (blue) was used for immunofluorescent counterstaining. Scale bars, 100 and 20 μm inaandb, respectively. Note that a cell cluster in the proximal posterior region from the otic vesicle (E) co-expresses GFP and tdTomato (left panel ina). In contrast, the majority of the GFP-positive cells are negative for tdTomato in a section of the distal posterior region of the otic vesicle (right panel). The bottom panel inbis a merged image from the top (GFP) and middle (tdTomato) panels and shows a high magnification view of GFP-tdTomato double-positive cells (arrows). (c–e) RT–qPCR analysis of the GFP-positive (+) and -negative (−) cell fractions that were sorted from the head and the liver regions of E9.5 (23–25 sp)22K-Epo-GFPtransgenic embryos. ‘T’ indicates unsorted total cells from the head region.EpoandGFPmRNA expression (c), neural crest marker (Wnt,Foxd3andSox10) mRNA expression (d) andAlbuminandEpoRmRNA expression (e) are shown as averages of relative expression levels with s.d. (n=5 in each group). The mRNA levels in the GFP-positive fractions from the head are set to 1 in each experiment after normalization usingGapdhmRNA expression levels. (f) The Epo concentrations in the culture supernatants of E8.5 embryonic organ. E8.5 embryonic organs (the head, heart and yolk sac (YS)) were incubated for 24 h under normoxic or hypoxic (1% oxygen) conditions. The Epo concentrations in the supernatants were measured using ELISA. The arrows indicate undetectable levels. The data were calculated from the levels of Epo that were produced by each organ from a given embryo and are reported (with s.d.) as the averages of the measurements from four embryos. Figure 4: A subpopulation of neural crest cells express the Epo gene. ( a , b ) Both GFP (green, arrowheads) and tdTomato (red) expression is detected in transverse sections of the neural tube (NT) from E9.5 17KXh-Epo-GFP:Wnt1-Cre:Rosa26R-tdTomato embryos using confocal microscopy. DAPI (blue) was used for immunofluorescent counterstaining. Scale bars, 100 and 20 μm in a and b , respectively. Note that a cell cluster in the proximal posterior region from the otic vesicle (E) co-expresses GFP and tdTomato (left panel in a ). In contrast, the majority of the GFP-positive cells are negative for tdTomato in a section of the distal posterior region of the otic vesicle (right panel). The bottom panel in b is a merged image from the top (GFP) and middle (tdTomato) panels and shows a high magnification view of GFP-tdTomato double-positive cells (arrows). ( c – e ) RT–qPCR analysis of the GFP-positive (+) and -negative (−) cell fractions that were sorted from the head and the liver regions of E9.5 (23–25 sp) 22K-Epo-GFP transgenic embryos. ‘T’ indicates unsorted total cells from the head region. Epo and GFP mRNA expression ( c ), neural crest marker ( Wnt , Foxd3 and Sox10 ) mRNA expression ( d ) and Albumin and EpoR mRNA expression ( e ) are shown as averages of relative expression levels with s.d. ( n =5 in each group). The mRNA levels in the GFP-positive fractions from the head are set to 1 in each experiment after normalization using Gapdh mRNA expression levels. ( f ) The Epo concentrations in the culture supernatants of E8.5 embryonic organ. E8.5 embryonic organs (the head, heart and yolk sac (YS)) were incubated for 24 h under normoxic or hypoxic (1% oxygen) conditions. The Epo concentrations in the supernatants were measured using ELISA. The arrows indicate undetectable levels. The data were calculated from the levels of Epo that were produced by each organ from a given embryo and are reported (with s.d.) as the averages of the measurements from four embryos. Full size image The GFP-positive cells in E9.5 17KXh-Epo-GFP embryos were separated with FACS, and the expressions of GFP reporter mRNA and endogenous Epo mRNA were examined using RT–qPCR. Consistent with the transgenic GFP expression, endogenous Epo mRNA expression was exclusively detected in the GFP-positive cell fraction of both the head and the liver regions ( Fig. 4c ; Supplementary Fig. S3a ). This result confirmed the faithful recapitulation of endogenous Epo gene expression by the 17KXh-Epo-GFP transgene. In the head region, the expression levels of the neural crest markers ( Wnt1, Foxd3 and Sox10 ) [31] , [32] , [33] were enriched in the GFP-positive cell fraction compared with the GFP-negative cell fraction ( Fig. 4d ). This indicates that a subpopulation of neural crest cells express the Epo gene. In contrast, very low-level expression of neural crest markers was observed in GFP-positive cells of the liver that expressed the Albumin gene, a hepatocyte marker ( Fig. 4d,e ). This result conclusively demonstrates that the Epo-expressing head cells are a different type of cells from Epo-expressing fetal hepatocytes [6] , [19] . Significant EpoR mRNA expression was detectable in GFP-negative head cells, which were circulating erythroid cells. Moreover, EpoR expression was strong in the GFP-negative liver cell fraction; the majority of these cells were definitive haematopoietic cells ( Fig. 4e ). When E8.5 embryos (5–9 sp) were dissected and each portion of the embryo was incubated for 24 h under normoxic or hypoxic (1% oxygen) conditions, we detected a significant concentration of Epo in the culture supernatant of the E8.5 head region, which contained GFP-positive cells. However, no Epo was observed in the supernatant from the heart or yolk sac regions ( Fig. 4f ). Epo production was not altered by hypoxic exposure of the neural tissue culture ( Fig. 4f ). These results demonstrate the consistency of GFP expression and Epo secretion in NEP cells. NEP cell-derived Epo induces primitive erythrocyte growth We then examined the activity of NEP cell-derived Epo by establishing a novel bioassay system ( Fig. 5a,b ). In this assay, we collected haematopoietic cells from yolk sacs of E8.5 Gata1-HRD (haematopoietic regulatory domain)-GFP transgenic mice, which contain GFP-positive primitive erythroid/megakaryocytic lineage cells [34] , [35] . The yolk sac cells were incubated with the dissected head region that contained NEP cells or heart region from E8.5 littermates without the transgene as a non-Epo-producing control. We performed cultures under hypoxic conditions (1% oxygen) to inhibit megakaryopoiesis, which is stimulated by ambient oxygen tension in yolk sac cell cultures [36] , [37] . 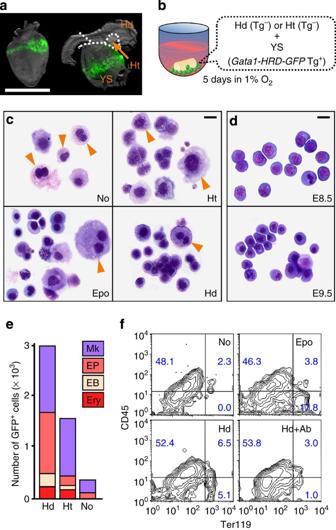Figure 5: NEP-derived Epo supports the growth of primitive erythroid cells. (a) GFP expression in aGata1-HRD-GFPtransgenic embryo at E8.5 (6 sp). The whole embryo with the yolk sac (left) was dissected into the yolk sac (YS), the head region (Hd) and the heart region (Ht). Scale bar, 1.0 mm. (b) A schematic representation of the strategy that was employed to investigate the bioactivity of the Epo produced by the neural crest cells. E8.5 embryos that were derived fromGata1-HRD-GFPtransgenic male and wild-type female mice were separated into GFP-expressing (Tg+) and -non-expressing (Tg−) embryos. The yolk sac cells of Tg+embryos were co-cultured with the Hd or Ht from a Tg–embryo in a 96-well round bottom plate for 5 days under 1% oxygen conditions. (c,d) Wright–Giemsa staining of cells that were derived from the yolk sac. Scale bars, 10 μm. The morphology of the cells that were incubated for 5 days (c) and of E8.5 (6 sp) and E9.5 (25 sp) primary cells before incubation (d) are shown. Note that whereas most cells from the culture with Epo or Hd are erythroblastic cells that stain dark purple, many megakaryoblastic cells (arrowheads) with multiple nuclei are observed in the cells that were incubated with Ht or without supplementation (No). (e) The total numbers of GFP-positive cells following a 5-day culture. The cultured cells were counted, and the expression levels of CD45, Ter119 and GFP were analysed using FACS. Mk, megakaryocytes (CD45−Ter119−); EP, erythroid progenitors (CD45+Ter119−); EB, erythroblast (CD45+Ter119+); Ery, mature erythrocytes (CD45−Ter119+). (f) The anti-Epo antibody blocks the effect of the Hd region on the differentiation of yolk sac cells. FACS analysis of GFP-positive cells was conducted with CD45 and Ter119 antibodies following 5 days of culture. The percentages of each quadrangle are given. ‘No’ indicates the control in which no supplementation was used. All the experiments were performed at least three times using more than four transgenic embryos, and representative data are presented. Figure 5: NEP-derived Epo supports the growth of primitive erythroid cells. ( a ) GFP expression in a Gata1-HRD-GFP transgenic embryo at E8.5 (6 sp). The whole embryo with the yolk sac (left) was dissected into the yolk sac (YS), the head region (Hd) and the heart region (Ht). Scale bar, 1.0 mm. ( b ) A schematic representation of the strategy that was employed to investigate the bioactivity of the Epo produced by the neural crest cells. E8.5 embryos that were derived from Gata1-HRD-GFP transgenic male and wild-type female mice were separated into GFP-expressing (Tg + ) and -non-expressing (Tg − ) embryos. The yolk sac cells of Tg + embryos were co-cultured with the Hd or Ht from a Tg – embryo in a 96-well round bottom plate for 5 days under 1% oxygen conditions. ( c , d ) Wright–Giemsa staining of cells that were derived from the yolk sac. Scale bars, 10 μm. The morphology of the cells that were incubated for 5 days ( c ) and of E8.5 (6 sp) and E9.5 (25 sp) primary cells before incubation ( d ) are shown. Note that whereas most cells from the culture with Epo or Hd are erythroblastic cells that stain dark purple, many megakaryoblastic cells (arrowheads) with multiple nuclei are observed in the cells that were incubated with Ht or without supplementation (No). ( e ) The total numbers of GFP-positive cells following a 5-day culture. The cultured cells were counted, and the expression levels of CD45, Ter119 and GFP were analysed using FACS. Mk, megakaryocytes (CD45 − Ter119 − ); EP, erythroid progenitors (CD45 + Ter119 − ); EB, erythroblast (CD45 + Ter119 + ); Ery, mature erythrocytes (CD45 − Ter119 + ). ( f ) The anti-Epo antibody blocks the effect of the Hd region on the differentiation of yolk sac cells. FACS analysis of GFP-positive cells was conducted with CD45 and Ter119 antibodies following 5 days of culture. The percentages of each quadrangle are given. ‘No’ indicates the control in which no supplementation was used. All the experiments were performed at least three times using more than four transgenic embryos, and representative data are presented. Full size image Following 5 days of incubation, we observed that more than half of the cells in the head region culture were morphologically erythroid cells ( Fig. 5c , Hd), which exhibited a small and mononuclear appearance that was similar to that of primitive erythroid cells that can normally be observed in E9.5 yolk sacs ( Fig. 5d ). These erythroid-lineage cells were predominant in the culture that was supplemented with recombinant Epo, and this culture condition was used as a positive control ( Fig. 5c , Epo). In contrast, no apparent stimulation of erythropoiesis was observed in the culture without supplementation ( Fig. 5c , No). In the co-culture with the heart region, megakaryocyte-like cells ( Fig. 5c , Ht, arrowheads) were increased in number, but erythroid cells were not. Using Gata1-HRD-GFP expression ( Supplementary Fig. S4 ), the primitive haematopoietic cells in the 5-day cultures were divided into four flow cytometric fractions: a CD45 − Ter119 − fraction containing megakaryocytes, a CD45 + Ter119 − fraction containing EP, a CD45 + Ter119 + fraction containing EBs and a CD45 − Ter119 + fraction containing mature erythrocytes (Ery) [38] . The number of Gata1-HRD-GFP-positive cells was ~10-fold higher in the culture with the head region than that in the control culture without supplementation ( Fig. 5e ). The number of Gata1-HRD-GFP-positive cells at the beginning of culture was estimated to be 500–1,000. Therefore, according to our previous finding that 10–20% of the 5,000 yolk sac cells at E8.5 were Gata1-HRD-GFP positive [35] , we estimated that a three- to sixfold increase in the number of Gata1-HRD-GFP-positive cells was induced during the 5-day culture with the head region. Although Gata1-HRD-GFP-positive cells were also increased in the culture with the heart region, the majority of the growing GFP-positive cells belonged to the megakaryocytic lineage ( Fig. 5e ). Recombinant Epo stimulates the maturation and anti-apoptosis activity of primitive erythrocytes in this culture system, and 17.8% of the GFP + cells were CD45 − Ter119 + Ery in the cultures that were supplemented with Epo ( Fig. 5f , Epo). In contrast, virtually no CD45 − Ter119 + cells were observed in the culture without supplementation ( Fig. 5f , No). In the culture with the head region, 5.1% of the cells were CD45 − Ter119 + ( Fig. 5f ; Hd), and the addition of a neutralizing antibody against Epo significantly inhibited erythroid differentiation ( Fig. 5f , Hd+Ab). These results demonstrate that NEP cells in the embryonic head region secrete functional Epo that can stimulate the proliferation and maturation of primitive erythroid cells. NEP cell-derived Epo stimulates erythroid cells in yolk sac Necessity of NEP cells for primitive erythropoiesis should be defined by NEP cell-specific deletion of the Epo gene. However, currently available Cre transgenic mouse lines are not suitable for the loss-of-function analyses of Epo secretion from NEP cells because only a small number of NEP cells are labelled in any of three mouse lines ( Wnt1-Cre , Pax3-Cre and P0-Cre ), which are known for Cre expression in neural crest cells (see Fig. 4 and Supplementary Fig. S3 ). We then hypothesized that Epo secreted from NEP cells reached the yolk sac through circulation to support the primitive erythropoiesis ( Fig. 6a ), as true heartbeats initiate around E9.0 (refs 7 , 8 ) and Epo-KO embryos exhibit abnormalities in the primitive erythropoiesis at this timing ( Fig. 1b,c ). To verify this hypothesis, we examined whether Epo from NEP cells reach the yolk sac and primitive erythroid cells are stimulated at E9.0. 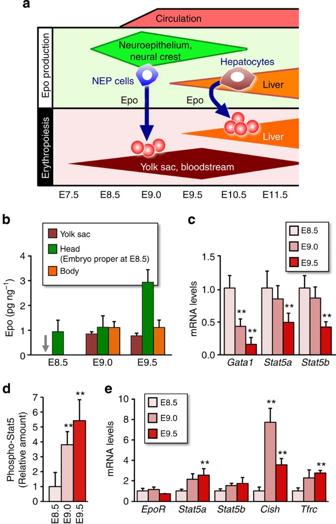Figure 6: NEP-derived Epo stimulates erythroid cells in the yolk sac through circulation. (a) A schematic model of the relationship between Epo-producing tissues and erythropoietic tissues during the ontogeny of mouse erythropoiesis. The first EPs emerge in the yolk sac at ~E7.5, and their maturation occurs in the yolk sac and the bloodstream. The first Epo production is initiated at E8.5 in NEP cells locating in the neural crest and the neuroepithelium. At ~E9.0, a true heartbeat can be observed, and NEP cell-derived Epo may stimulate erythroid cells in the yolk sac through the bloodstream. After E9.5, the hepatocytes begin to produce Epo for erythroid cells in the fetal liver. Note that secreted Epo from NEP cells seems to support the growth of erythroid cells in an endocrine manner before the erythropoietic site moves to the liver. (b) Amounts of Epo protein in the indicated parts of embryos at E8.5 (6–9 sp), E9.0 (16–20 sp) and E9.5 (22–25 sp) were measured by ELISA. Dissection of embryos was carried out as described inSupplementary Fig. S2a–c. Data were presented as the averages of four groups of pooled samples from more than five embryos after normalization with the total protein amount. The Epo amount in E8.5 YS was undetectable (arrow). (c–e) Changes in mRNA expression profiles and in phospho-Stat5 amounts from E8.5 to E9.5 in the yolk sac. Relative expression levels ofGata1,Stat5aandStat5bmRNAs in the yolk sac were determined after normalization with theGapdhmRNA expression levels (c). Relative amounts of phospho-Stat5 in a yolk sac were measured and calculated by ELISA using the phosphorylated Stat5(Y699)-specific antibody (d). mRNA levels of the indicated genes in the yolk sac erythroid cells are represented after normalization with theGata1mRNA expression levels to be compensated by erythroid population in the yolk sac (e). Data from E8.5 samples is set to 1, and the data are shown as the averages of four to six samples with s.d. (c–e). **P<0.01 when compared with the E8.5 samples based on Student’st-test (c–e). Figure 6: NEP-derived Epo stimulates erythroid cells in the yolk sac through circulation. ( a ) A schematic model of the relationship between Epo-producing tissues and erythropoietic tissues during the ontogeny of mouse erythropoiesis. The first EPs emerge in the yolk sac at ~E7.5, and their maturation occurs in the yolk sac and the bloodstream. The first Epo production is initiated at E8.5 in NEP cells locating in the neural crest and the neuroepithelium. At ~E9.0, a true heartbeat can be observed, and NEP cell-derived Epo may stimulate erythroid cells in the yolk sac through the bloodstream. After E9.5, the hepatocytes begin to produce Epo for erythroid cells in the fetal liver. Note that secreted Epo from NEP cells seems to support the growth of erythroid cells in an endocrine manner before the erythropoietic site moves to the liver. ( b ) Amounts of Epo protein in the indicated parts of embryos at E8.5 (6–9 sp), E9.0 (16–20 sp) and E9.5 (22–25 sp) were measured by ELISA. Dissection of embryos was carried out as described in Supplementary Fig. S2a–c . Data were presented as the averages of four groups of pooled samples from more than five embryos after normalization with the total protein amount. The Epo amount in E8.5 YS was undetectable (arrow). ( c – e ) Changes in mRNA expression profiles and in phospho-Stat5 amounts from E8.5 to E9.5 in the yolk sac. Relative expression levels of Gata1 , Stat5a and Stat5b mRNAs in the yolk sac were determined after normalization with the Gapdh mRNA expression levels ( c ). Relative amounts of phospho-Stat5 in a yolk sac were measured and calculated by ELISA using the phosphorylated Stat5(Y699)-specific antibody ( d ). mRNA levels of the indicated genes in the yolk sac erythroid cells are represented after normalization with the Gata1 mRNA expression levels to be compensated by erythroid population in the yolk sac ( e ). Data from E8.5 samples is set to 1, and the data are shown as the averages of four to six samples with s.d. ( c – e ). ** P <0.01 when compared with the E8.5 samples based on Student’s t -test ( c – e ). Full size image We analysed Epo levels in the embryonic parts using enzyme-linked immunosorbent assay (ELISA). Consistent with the above RT–qPCR results ( Fig. 2a ; Supplementary Fig. S5 ), we detected significant concentrations of Epo in the embryo proper at E8.5, and in the head regions at E9.0 and E9.5 ( Fig. 6b ). In the yolk sac, while Epo was below the detectable level at E8.5, Epo started reaching the yolk sac after E9.0 and became detectible ( Fig. 6b ). These results are consistent with NEP cells in the head region beginning to produce Epo at E8.5, and the Epo being delivered into yolk sac through the blood flow after E9.0 when the circulatory system is activated [7] , [8] . We next examined downstream pathway of the Epo-EpoR system in the yolk sac. Gata1 mRNA level was decreased in the yolk sac from E8.5 to E9.5, when the level was normalized with the housekeeping Gapdh mRNA level ( Fig. 6c ), suggesting that the ratio of erythroid cells decreased in the yolk sac that is rapidly expanding during these embryonic stages [35] . The expression of Stat5 genes ( Stat5a and Stat5b ) was detected at E8.5 and the levels were decreased at E9.0 and E9.5, similar to the Gata1 gene expression ( Fig. 6c ). In contrast, phosphorylated Stat5 level was very low at E8.5 but the amount in each yolk sac was significantly increased after E9.0 ( Fig. 6d ). Since Epo-binding to EpoR immediately induces phosphorylation and transcriptional activity of Stat5 (ref. 39 ), these results are consistent with NEP cell-derived Epo activating the primitive erythropoiesis at E9.0. We also found that the Cish gene, one of the early response genes to Epo stimulation [2] , [21] , was dramatically induced at E9.0 ( Fig. 6e ). The gene for CD71 ( Tfrc ), which is known as a target of Stat5 (ref. 39 ), was also upregulated after E9.0, showing a very good agreement with the decreased expression level of CD71 in yolk sac of E9.0 Epo-KO embryos ( Fig. 1c ). These results are thus consistent with NEP cell-derived Epo reaching EpoR on the yolk sac erythroid cells through the bloodstream after E9.0, and inducing Stat5 activation and expressions of the Cish and Tfrc genes ( Supplementary Fig. S6 ). Since NEP cells are the only source of Epo in E9.0 embryos ( Supplementary Fig. S5 ), it is possible to think that defects in the primitive erythropoiesis of Epo-KO embryos at E9.0 ( Fig. 1b,c ) are provoked by the loss of Epo production in NEP cells. Although Epo or EpoR deficiency appears to affect primitive erythropoiesis, the roles that Epo plays in primitive erythropoiesis or the cells that supply Epo for primitive erythropoiesis have not been elucidated. As summarized in Fig. 6a , in the present study we demonstrate that Epo is indeed required for the progression of primitive erythropoiesis in mouse embryos. We further have discovered that a major source of Epo for primitive erythropoiesis might be a subpopulation of neural and neural crest cells, which we refer to as NEP cells. Consistent with our observation, the principal Epo-producing tissue in zebrafish larvae is neural tissue, and Epo production moves to the heart and liver during adulthood [40] , [41] . We also observed that a subpopulation of NEP cells migrate along the blood vessels in the intersomitic space. It therefore appears that NEP cell-derived Epo may efficiently stimulate the differentiation of primitive erythroid cells in the yolk sac and bloodstream (see Fig. 6a ). Indeed, defects in the heartbeat of mouse embryos cause the maturation arrest of primitive erythroid cells [42] . These results firmly support the contention that NEP cells support primitive erythropoiesis in the yolk sac. CD71, a transferrin receptor, plays important roles in iron uptake for haemoglobin synthesis [43] . As CD71 expression in primitive EBs is reduced significantly after E9.0 in Epo-deficient mice, Epo appears to be indispensable for the CD71 expression and late-stage primitive erythropoiesis. The CD71 expression is also impaired in the definitive erythroid cells of EpoR-deficient mice [17] , indicating that the Epo signal is essential for the upregulation of CD71 expression during erythroid maturation in both primitive and definitive erythropoiesis. The loss of Stat5, an important transcription factor in the Epo signalling cascade, in definitive erythroid cells causes the downregulation of CD71 expression [39] . Thus, our finding that CD71 expression is decreased in primitive erythroid cells of Epo-KO embryos suggests that the Epo-mediated induction of CD71 expression via Stat5 activation may play an indispensable role in primitive erythroid cells. The neural crest is considered to be the fourth germ layer of vertebrates. The neural crest appears transiently in embryos at the mid-gestational stage, and neural crest cells differentiate into a variety of cell types, including neuronal, cardiac and skeletal cells [27] , [31] . Many studies have sought to delineate the nature of the neural crest cells and their derivatives, including studies in avian embryos. However, many aspects of mammalian neural crest cells that are related to cell fate and other properties remain unknown. This study provides evidence that a subpopulation of mouse neural crest cells, which express Wnt1 , Foxd3 and Sox10 , produce Epo. In this regard, the origin of the REP cells is an intriguing question and remains unknown [20] . REP cells express the interstitial fibroblast marker CD73 and neuronal markers, such as microtubule-associated protein 2 and neurofilament light polypeptide [19] , [20] , [21] , [44] , [45] . Neural crest-derived cells distribute in the interstitial space of renal tubules in adult mice [45] . These observations support the notion that REP cells are derived from neural crest cells. This hypothesis is further supported by the similarity in the regulatory mechanisms for the Epo gene in NEP and REP cells. Epo gene expression levels in both NEP and REP cells do not require the GATA motif or the HIF-binding motif, both of which are essential for the regulation of Epo in hepatocytes [6] , [19] . Several reports have demonstrated that the Epo-EpoR signalling plays important roles in non-haematopoietic cells, including neuronal and cardiac cells [11] , [12] , [13] . To address the non-haematopoietic roles of Epo, we have developed a mouse line that expresses EpoR only in haematopoietic cells; however, these mice exhibit no apparent abnormality during embryogenesis [17] . We have also observed that Epo-KO embryos exhibit no apparent abnormality until E11.5 in non-haematopoietic organs. In zebrafish, the overexpression and knockdown of Epo dramatically alter erythropoiesis in the embryonic intermediate cell mass and the adult kidney, but these alterations in Epo levels do not affect the development of non-haematopoietic systems [41] . Moreover, NEP cells express low EpoR mRNA levels compared with haematopoietic cells. On the basis of these observations, we conclude that NEP cell-secreted Epo is dispensable for the morphogenesis of non-haematopoietic tissues and for the migration of neural and neural crest cells. In summary, we have determined that a subpopulation of neural cells and a subpopulation of neural crest cells produce Epo to support primitive erythropoiesis during ontogeny. Of the many important issues that remain to be clarified, the following two are particularly intriguing. One is whether Epo signalling is required for the stress response of embryonic tissues, as observed in adult tissues. Another is whether neural crest-derived cells in adults have the potential to produce Epo in response to anaemic stress conditions. Further studies are necessary to elucidate the nature of NEP cells and the contributions of NEP cell-derived Epo to embryonic haematopoiesis. Mice We previously established the Epo-deficient mouse line in which enhanced GFP complementary DNA (BD Biosciences) was inserted into the Epo locus [20] , [21] . The Epo-GFP transgenic mouse lines and the Gata1-HRD-GFP transgenic mouse line were also previously generated [6] , [15] , [19] , [22] , [34] . The 17KXh-Epo-GFP transgene contains the upstream 17-kb and downstream 15-kb sequences of the Epo gene ( Supplementary Fig. S1 ). The 5′-GATA (5′-TGATAA-3′) motif in the wt-Epo-GFP construct was mutated to 5′-T T ATAA-3′ and 5′-T TT TAA-3′ in the m1-Epo-GFP and the m2-Epo-GFP constructs, respectively [19] . The m3-Epo-GFP transgene has a mutation in the 3′-HRE (from 5′-ACGTG-3′ to 5′-A AAA G-3′) [6] . To trace the neural crest cells, Rosa26R-tdTomato mice [46] were crossed with Wnt1-Cre [28] , Pax3-Cre [29] or P0-Cre [30] transgenic mouse lines, all of which except P0-Cre mice (the Kumamoto University) were supplied by Jackson Laboratory. The genotype of these mice was determined using genomic PCR analysis with the primers that are listed in Supplementary Table S1 . The animal experiments were performed according to the Regulations for Animal Experiments and Related Activities of Tohoku University and the regulations of the Standards for Human Care and Use of Laboratory Animals of the University of Tsukuba. Flow cytometry and cell sorting For the cell surface marker analyses, single-cell suspensions of yolk sacs were prepared by passing the cells through a needle. Antibody-stained cells were also stained with propidium iodide to gate out dead cells and were analysed using a FACS. We used the FACSCalibur with CellQuest programme (Becton Dickinson). For the cell sorting analysis, single-cell suspensions were prepared by digesting embryonic tissues with Trypsin-EDTA (0.05%, Invitrogen) for 30 min at 37 °C. The GFP-positive cells were sorted using FACSVantage SE and FACSAria II (Becton Dickinson). The mean fluorescent intensity and the percentage of the normal distribution of the GFP + and GFP − fractions were calculated. The phycoerythrin-conjugated anti-Ter119, allophycocyanin-conjugated anti-CD71 antibodies, allophycocyanin-conjugated anti-CD45 antibodies were obtained from BD Biosciences and used at 1:100 dilution. RT–qPCR The RNA samples were purified from dissected embryonic organs and FACS-sorted cells using the RNeasy kit (Qiagen). The total RNA was reverse transcribed using SenscriptRT (Qiagen). For the RT–qPCR analyses, Epo mRNA levels were measured using the ABI PRISM 7300 or StepOne real-time PCR systems (Applied Biosystems). Gapdh mRNA was used as an internal standard [6] , [19] . All primer sequences are listed in Supplementary Table S1 . Histological analyses The fluorescence of transgenic embryos was observed using a MZ16FA microscope (Leica) and a LMS510 confocal imaging system (Carl Zeiss). For the immunohistochemical analyses, the embryos were fixed in 4% paraformaldehyde for 15 min. Frozen sections (25 μm thickness) were collected from the fixed embryos after embedding them in blocks of OCT (Sakura Finetechnical). The following antibodies were used for the immunohistochemical analyses: anti-GFP rabbit polyclonal antibody (Medical & Biological Laboratories, 1:500 dilution), anti-CD31 rat monoclonal antibody (e-Bioscience, 1:100 dilution), anti-Sox2 rabbit polyclonal antibody (Abcam, 1:1000 dilution) and Alexa fluor 488- or 555-conjugated secondary antibodies (Molecular Probes, 1:500 dilution). Epo bioassay GFP-expressing yolk sacs were selected from E8.5 littermates that were obtained from the mating of Gata1-HRD-GFP transgenic male mice [31] with wild-type female mice. Single-cell suspensions were prepared from the yolk sacs by incubating them in 0.05% Trypsin-EDTA (Invitrogen) for 5 min. Five thousand cells were incubated in 0.1 ml RPMI medium (Sigma) that was supplemented with 10% fetal bovine serum (Hyclone), 2-mercaptoethanol (0.1 mM) and antibiotics. The incubations were performed with or without human recombinant Epo (4 mU ml −1 , Chugai Pharmaceutical) in 96-well round bottom plates in a multi-gas incubator (Astec) at 5% CO 2 and 1% O 2 . GFP-negative embryos from the same litters were dissected as shown in Supplementary Fig. S2a and added to these yolk sac cell cultures. An anti-Epo antibody (10 μg ml −1 , R&D Systems) was used to block Epo function in the culture medium. Following a 5-day incubation, the cells were harvested by pipetting and the GFP-expressing cells were analysed. ELISA To measure Epo concentrations in mouse embryonic parts, mouse embryos were dissected as shown in Supplementary Fig. S2a–c , and the dissected parts from more than five embryos were gathered into a sampling tube. The pooled samples were lysed by pipetting after two freeze-thaw cycles and Epo amount was measured using a mouse Epo ELISA kit (R&D Systems). Total protein amount of the lysate was measured using the Bradford assay (Bio-Rad). To measure the Epo secretion, the dissected organs ( Supplementary Fig. S2a ) from four embryos were pooled into 0.1 ml of RPMI medium (Sigma) that was supplemented with 10% fetal bovine serum (Hyclone). After 24-h incubation under normoxic or hypoxic (1% O 2 ) conditions at 37 °C, the supernatants were measured the Epo concentrations using a mouse Epo ELISA Kit. For ELISA of phosphorylated Stat5, a single-cell suspension of the yolk sac, which was prepared by pipetting, was fixed by 8% formaldehyde on the 96-well plate under a centrifuging condition (500 g ) for 20 min at room temperature. The relative amounts of phospho-Stat5 in each yolk sac were analysed using a rabbit anti-Stat5(Y699) antibody from cell-based ELISA system (R&D Systems) following the instruction manual. How to cite this article: Suzuki, N. et al. Erythropoietin production in neuroepithelial and neural crest cells during primitive erythropoiesis. Nat. Commun. 4:2902 doi: 10.1038/ncomms3902 (2013).